Aromatic porous-honeycomb electrodes for a sodium-organic energy storage device Rechargeable batteries using organic electrodes and sodium as a charge carrier can be high-performance, affordable energy storage devices due to the abundance of both sodium and organic materials. However, only few organic materials have been found to be active in sodium battery systems. Here we report a high-performance sodium-based energy storage device using a bipolar porous organic electrode constituted of aromatic rings in a porous-honeycomb structure. Unlike typical organic electrodes in sodium battery systems, the bipolar porous organic electrode has a high specific power of 10 kW kg −1 , specific energy of 500 Wh kg −1 , and over 7,000 cycle life retaining 80% of its initial capacity in half-cells. The use of bipolar porous organic electrode in a sodium-organic energy storage device would significantly enhance cost-effectiveness, and reduce the dependency on limited natural resources. The present findings suggest that bipolar porous organic electrode provides a new material platform for the development of a rechargeable energy storage technology. Next-generation rechargeable batteries are key devices for the successful development of green technologies [1] , for example, a grid system combined with large-scale storage and renewable energy, and electric vehicles. Currently, rechargeable lithium batteries are the leading candidate for such utilizations. However, abundance of commercially viable lithium source is low, which may be detrimental to future costs and energy supply stability. In spite of this, there is a huge demand for lithium batteries to be used in a variety of devices, for example, portable electronic devices and electronic vehicles [1] , [2] , [3] , [4] , [5] , [6] . A key issue for successfully developing green technologies is affordability. There is an urgent need for alternative energy storage devices with a performance comparable to, or better than rechargeable lithium batteries. One possible approach is to use sodium as an alternative charge carrier [3] , [4] , [5] , [6] , [7] , [8] , [9] , [10] , [11] , [12] , [13] , [14] , [15] , [16] , [17] , [18] to lithium, as the cost of sodium carbonate (Na 2 CO 3 ), for example, is only 3% of Li 2 CO 3 (ref. 5 ). Another even more effective approach to improving affordability is to replace the current metal-based electrodes with organic materials [19] , [20] , [21] , [22] , [23] , [24] , [25] , [26] , [27] that are more abundant in nature. Since the advent of conductive polymers [28] and reversible redox polymers [22] , a large number of p -, n - and bipolar organic electrodes have been investigated for energy storage devices due to their low-cost and possible applications in flexible plastic batteries [21] . Although there is a long history of research in sodium-based energy storage devices, there have been only a few reports of organic materials applied to rechargeable sodium batteries, for example, polyparaphenylene and sodium terephthalate [23] , [24] , [27] , and often they are only suitable as the anode. Finding a new, suitable group of organic materials for use as cathodes in sodium batteries could stimulate the development of sodium-based energy storage devices and meet the requirement of next-generation batteries, namely high-specific energy and power, and most importantly, affordability. We report bipolar porous polymeric frameworks as a new class of affordable organic electrodes for a sodium-based energy storage device: an aromatic porous-honeycomb cathode, which shows a long cycle life of over 7,000 cycles and performances comparable to lithium-ion batteries, which are a high-specific power of 10 kW kg −1 and a specific energy of 500 Wh kg −1 based on the weight of the organic electrode in half-cells. Physical characterization of the porous organic electrode The bipolar porous organic electrode (BPOE) is a porous-honeycomb, polymeric framework consisting of benzene rings and triazine rings in two-dimensional (2D) structure ( Fig. 1a ) [29] , [30] . Using high-resolution transmission electron microscopy, we have confirmed that the BPOE has a sheet-like morphology, which is with ~300 nm wide ( Fig. 1b ) and typically we observed <10 stacking layers, giving a thickness of ~4 nm ( Fig. 1b inset). Raman spectroscopy ( Fig. 1c ), Fourier-transform infrared (FT-IR) spectroscopy ( Supplementary Fig. S1 ) and X-ray diffractometry ( Supplementary Fig. S2 ) gives a further details about the BPOE: This framework is formed as a short-range-ordered 2D structure with the stacking of each 2D unit ( Fig. 1a ) in a non-coplanar fashion [29] , [30] , [31] as the global structure. Raman spectroscopy measurements (RSMs) allow to reveal the electronic structure of materials (=information about a structural periodicity of a material) [32] , [33] , [34] . Especially, graphite and graphene have been extensively researched concerning their electronic structure by RSMs [32] , [33] , [34] , [35] , [36] . The G peak is produced by the doubly degenerated zone centre E 2 g mode, which is a motion of atoms in the 2D honeycomb structure [32] , [33] , [34] . This G peak also appears in the porous-graphene at same position, as well as graphene. Furthermore, carbon nitride formed in 2D honeycomb structure shows the G peak at ~1,600 cm −1 (refs 35 , 36 ). Therefore, the G peak at ~1,600 cm −1 in Fig. 2c reveals the existence of a 2D porous-honeycomb structure, which is constituted by benzene rings and triazine rings. This structure, which is revealed by Raman spectroscopy, FT-IR spectroscopy and X-ray diffractometry, is comparable to hard carbon, a disordered carbon consisting of single graphene sheets stacked at random angles [37] . Electron energy-loss spectroscopy measurements show a 1s→π* transition, which reveals the sp 2 -hybridization for carbon and nitrogen at 285 eV and 400 eV, respectively, ( Fig. 1d ) and the fine structure of the C- K and N- K edges also suggest a graphitic network with sp 2 -bonding [38] . Indeed, we investigated the porous structure of the BPOE by nitrogen physisorption experiments ( Fig. 2a ). Its pore-size distribution confirmed the existence of micropores of ca.1.4 nm ( Fig. 1a ), which was observed by previous reports [29] , [30] , [31] ( Fig. 2b ). From these measurements, we confirmed the formation of a short-range-ordered 2D polymeric framework constituted by aromatic rings. Therefore, the BPOE shows adjustable electronic properties and controllable semiconducting features emerging from their structural periodicity comparable to 2D atomic crystals, such as multilayer graphene, and a choice of monomer as a building block [39] , [40] , [41] , [42] , [43] , [44] , [45] . Here we demonstrate that the bipolar characters of the BPOE required for high-performance electrochemical properties are preserved even in a sodium battery system. 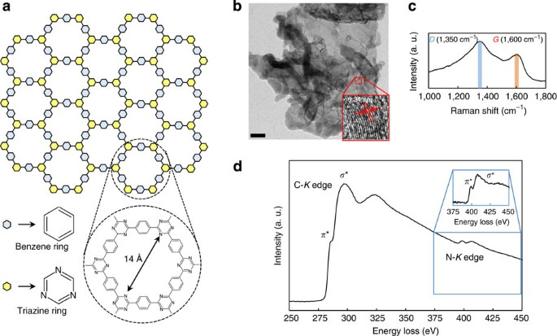Figure 1: Structure and spectroscopy measurements for BPOE. (a) Schematic illustration of the ideal BPOE having a porous-honeycomb structure with a pore diameter of 14 Å. The 2D structure of the BPOE is constituted by triazine rings and benzene rings. (b) Transmission electron microscopy image of the BPOE showing a sheet-like morphology. The scale bar indicates 100 nm. The inset shows a cross-section of a multilayer BPOE, stacking of about 10 layers. (c) Raman spectrum of the BPOE at a laser excitation of 632.8 nm. The existence of theGpeak reveals the graphene-like 2D structure. (d) Electron energy-loss spectrum of the carbon and nitrogenKedges recorded in the BPOE. The inset shows the N-Kedge with subtraction of the background. The existence ofsp2-hybridized carbon and nitrogen atoms reveals the formation of graphitic network constituted by triazine and benzene rings. a.u., arbitrary unit. Figure 1: Structure and spectroscopy measurements for BPOE. ( a ) Schematic illustration of the ideal BPOE having a porous-honeycomb structure with a pore diameter of 14 Å. The 2D structure of the BPOE is constituted by triazine rings and benzene rings. ( b ) Transmission electron microscopy image of the BPOE showing a sheet-like morphology. The scale bar indicates 100 nm. The inset shows a cross-section of a multilayer BPOE, stacking of about 10 layers. ( c ) Raman spectrum of the BPOE at a laser excitation of 632.8 nm. The existence of the G peak reveals the graphene-like 2D structure. ( d ) Electron energy-loss spectrum of the carbon and nitrogen K edges recorded in the BPOE. The inset shows the N- K edge with subtraction of the background. The existence of sp 2 -hybridized carbon and nitrogen atoms reveals the formation of graphitic network constituted by triazine and benzene rings. a.u., arbitrary unit. 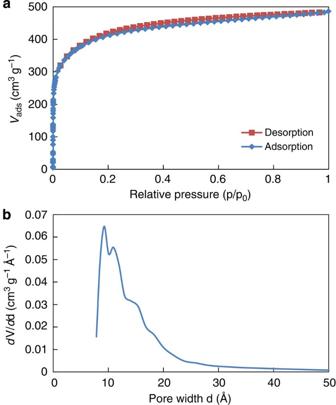Figure 2: Pore structure of the BPOE. (a) Results of nitrogen physisorption experiments for the BPOE. (b) Pore-size distribution of the BPOE. Full size image Figure 2: Pore structure of the BPOE. ( a ) Results of nitrogen physisorption experiments for the BPOE. ( b ) Pore-size distribution of the BPOE. Full size image Electrochemical characterizations of the BPOE Electrochemical impedance spectroscopy (EIS) measurements were carried out at 3.3 V versus Na/Na + ( p -doping process, Fig. 3a ) and 2.3 V versus Na/Na + ( n -doping process, Fig. 3c ) after achieving each quasi-equilibrium state [46] in order to probe the physical and/or chemical phenomena at the interface between the BPOE and the electrolyte solution. A frequency range of 10 mHz–10 kHz with an amplitude of 10 mV was applied in all EIS measurements. The Nyquist plots obtained by the EIS measurements were fitted using an equivalent circuit based on the Randels model [29] , [47] showing in Fig. 3a , where R is the electrolyte resistance, CPE={ T CPE ( jω ) α } –1 is a constant phase element with ω being the angular frequency and α an empirical electrode roughness parameter, and where Z w is the Warburg impedance indicating a diffusion-limited electrochemical reaction. Each Nyquist plot above and below 2.8 V versus Na/Na + shows a semicircle at high frequencies suggesting charge transfer at the polymeric framework/electrolyte (1 M NaClO 4 in propylene carbonate (PC)) interface and a characteristic linear diffusion-limited response at a tilt angle of close to 45° at low frequencies indicating incorporation of the ion in the electrode materials [17] , [29] , [47] . The FT-IR and RSMs ( Fig. 3e ) confirmed the coordination of the anion (ClO 4 – ) in the polymeric framework, which was electrochemically incorporated. The ClO 4 − doped BPOE is indicated as I; 1 M NaClO 4 in PC is indicated as II; and PC is indicated as III. In Fig. 3e , which shows the Raman spectra, the peaks assigned 1 originate from PC. The peak 2A in II (935 cm −1 ) is the infrared-inactive, but is Raman-active ν 1 mode for free ClO 4 – (refs 48 , 49 , 50 ). This Raman-active ν 1 mode and the signals form PC were not detected for I, which means that there is no residual electrolyte in I. In Fig. 3f , which shows the FT-IR spectra, the peak 2B in I (881 cm −1 ) is the infrared-active ν 1 mode for ClO 4 – (refs 48 , 51 ). The infrared-inactive ν 1 mode becomes infrared-active due to destruction of the symmetry by the coordination to host compounds. In our case, the destruction of the symmetry is induced by the electrochemical p -doping, which creates a coordination of ClO 4 – to the BPOE. The peaks assigned 1′ in II and III ( Fig. 3f ) originate from PC. The peak 3 in I ( Fig. 3f ) can be assigned to aromatic C–H out-of-plane bend or 1,4-disubstituted benzene rings in the BPOE (ref. 29 ). From these spectroscopy measurements, the doped ClO 4 – state in the BPOE was observed. Thus, the results of the FT-IR and RSMs clearly reveal the successful p -doping of ClO 4 – in the BPOE. Based on this bipolar feature of the BPOE, we can achieve a large working potential window (4.1–1.3 V versus Na/Na + ), which can increase the energy density by giving a high-specific capacity. Moreover, its porous morphology results in a high rate capability due to fast ion-transport by the electrolyte filled porous framework ( Fig. 2a ). 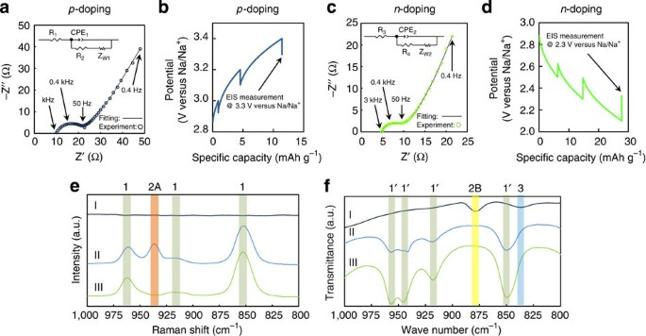Figure 3: Electrochemical characteristics of the BPOE. (a) Typical Nyquist plot in thep-dopable region and its equivalent circuit.R1=10.53 Ω,R2=8.51 Ω,TCPE1=437.16 μF, andα=0.91. (b) Potential value at the quasi-equilibrium state for the EIS measurement in thep-dopable region. (c) Typical Nyquist plot in then-dopable region and its equivalent circuit.R3=4.82 Ω,R4=3.15 Ω,TCPE2=154.13 μF, andα=0.92. (d) Potential value at the quasi-equilibrium state for the EIS measurement in then-dopable region. (e) RSMs for the ClO4−doped BPOE (indicated as I), 1 M NaClO4in PC (indicated as II), and PC (indicated as III). (f) FT-IR measurements for I, II and III. (a.u. refers to arbitrary unit). Figure 3: Electrochemical characteristics of the BPOE. ( a ) Typical Nyquist plot in the p -dopable region and its equivalent circuit. R 1 =10.53 Ω, R 2 =8.51 Ω, T CPE1 =437.16 μF, and α =0.91. ( b ) Potential value at the quasi-equilibrium state for the EIS measurement in the p -dopable region. ( c ) Typical Nyquist plot in the n -dopable region and its equivalent circuit. R 3 =4.82 Ω, R 4 =3.15 Ω, T CPE2 =154.13 μF, and α =0.92. ( d ) Potential value at the quasi-equilibrium state for the EIS measurement in the n -dopable region. ( e ) RSMs for the ClO 4 − doped BPOE (indicated as I), 1 M NaClO 4 in PC (indicated as II), and PC (indicated as III). ( f ) FT-IR measurements for I, II and III. (a.u. refers to arbitrary unit). Full size image In Fig. 4a , we show the charge–discharge curves for the BPOE in a rechargeable sodium battery system at various current densities ranging from 0.01 Ag –1 to 5.0 Ag –1 in a working potential of 1.3–4.1 V versus Na/Na + . These curves were then compared with open-circuit voltage (OCV) curves obtained by using the galvanostatic intermittent titration technique ( Supplementary Fig. S3 ). This sloping nature of the charge–discharge curves could be related to the 2D structure and defects due to the short-range-ordered structure of the BPOE, which results in a different electronic structure compared with the bulk material and affects the electrochemical properties [52] , [53] , [54] . The initial OCV is ~2.8 V versus Na/Na + , and therefore, the p -dopable and n -dopable regions are above and below 2.8 V versus Na/Na + , respectively. We used 1 M NaClO 4 in PC as an electrolyte due to its high stability in the Na-ion battery system [16] . For a high current density of 5 A g –1 , the BPOE can provide a specific capacity of ~50 mAh g –1 . To calculate the approximate values for the doping of Na + and ClO 4 – , we refer to a trimerized p -dicyanobenzene (molecular weight of 384.09 g mol –1 , here referred to as C 3 N 3 ) as the unit cell of the BPOE. 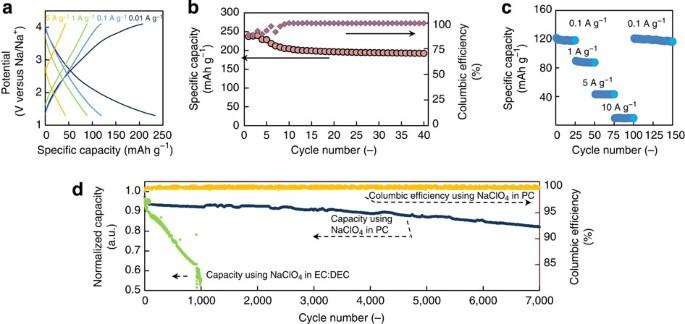Figure 4: Cycle performance and rate capability of the BPOE. (a) Charge–discharge curves of a sodium-organic energy storage device at various current densities. (b) Cycle performance of a sodium-organic energy storage device at a current density of 0.01 A g−1. (c) Cycle performance of a sodium-organic energy storage device under harsh conditions. (d) Cycle performance of a sodium-organic energy storage device up to 7,000 cycles with comparing the effect of electrolytes. The two redox reactions can then be defined as Figure 4: Cycle performance and rate capability of the BPOE. ( a ) Charge–discharge curves of a sodium-organic energy storage device at various current densities. ( b ) Cycle performance of a sodium-organic energy storage device at a current density of 0.01 A g −1 . ( c ) Cycle performance of a sodium-organic energy storage device under harsh conditions. ( d ) Cycle performance of a sodium-organic energy storage device up to 7,000 cycles with comparing the effect of electrolytes. Full size image for a potential range of 4.1–2.8 V versus Na/Na + : that is, the p -dopable region, and for the potential range of 2.8–1.3 V versus Na/Na + : that is, n -dopable region. A discharge capacity of 55 mAh g –1 ( p -undoping) was obtained at a very-low current density of 0.01 Ag –1 ( Fig. 4a ) for equation (1) in the p -dopable region (>2.8 V versus Na/Na + ), resulting in x =0.79 from equation (1) and a specific discharge capacity of 185 mAh g –1 ( n -doping) was obtained ( Fig. 4a ) for equation (2) in n -dopable region (<2.8 V versus Na/Na + ), yielding y =2.65 from equation (2). The big difference of the discharge capacity for the p -undoping and the n -doping process could come from the different energy storage mechanism: if we compare the rate capability of the p -undoping and n -doping processes ( Supplementary Table S1 ), the p -undoping process shows a better rate performance compared with the n -doping process. This result indicates that the storage mechanism for the p -doping/-undoping process (the storage reaction related to ClO 4 – ) could occur at the surface of the BPOE, which is like a pseudo-Faradaic reaction showing a capacitive behaviour. And the n -doping/-undoping process is suggested that it could be an insertion/de-insertion of Na + into the BPOE, which is a Faradaic reaction. Cycle performance and rate capability of the BPOE The cycle performance of the BPOE was checked at a range current densities, from a very-low current density of 0.01 A g –1 up to a high current density of 5.0 A g –1 revealing quite good cycle stability ( Fig. 4a–c ): At a current density of 0.01 A g –1 , the BPOE shows a specific capacity of ~200 mAh g –1 based on the mass of the BPOE and a stable cycle performance ( Fig. 4b ). Even under harsh conditions (25 cycles at different current densities from 0.1 A g –1 to 5.0 A g –1 without relaxation between the cycles), the BPOE reproduces a stable-specific capacity of ~120 mAh g –1 at 0.1 A g –1 , retaining the same specific capacity as in the first 25 cycles at 0.1 A g –1 ( Fig. 4c ). Moreover, BPOE has been tested over 7,000 cycles with 80% capacity retention at a high current density of 1.0 A g –1 ( Fig. 4d ). Raman spectra of the electrode after 7,400 charge–discharge cycles provide further evidence of the stability of the 2D framework by showing the G peak ( Supplementary Fig. S4 ). The importance of the selection of the electrolyte is evident by comparing two different electrolytes for the cycle stability test. Both 1 M NaClO 4 in ethylene carbonate (EC): diethyl carbonate (DEC) (1:1) and 1 M NaClO 4 in PC were reported as stable electrolytes for the Na-ion battery system up to 100 cycles [16] . In contrast to 1 M NaClO 4 in PC, the cell with 1 M NaClO 4 in EC:DEC begins to show a degradation from about 200 cycles. The reason for the performance degradation may be due to a reaction of the BPOE with the organic solvents and Na + ; solid products that were observed to form on the counter electrode (Na metal) for the cells, which used 1 M NaClO 4 in EC:DEC as electrolyte ( Supplementary Fig. S5 ). This dramatic difference in cycling stability suggests that PC is one of the most stable organic solvents for Na-ion battery systems of this configuration. Energy storage principle of the BPOE In Fig. 5a–c , we show the discharge process based on the energy storage principle of a BPOE. The unique points of the BPOE are: (1) this material can be used as a cathode, (2) BPOE is a bipolar material, which has a p -dopable region above the initial OCV and a n -dopable region below the initial OCV and (3) its p -undoping process ( Fig. 5a ) and n -doping process ( Fig. 5b ) can be continuously and linearly connected [29] ( Fig. 5c ). Therefore, we can expect a higher energy density from the BPOE due to a wide working potential compared with a material having only the p - or n -dopable property. 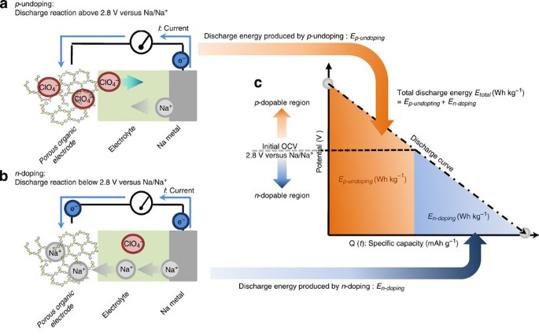Figure 5: Energy storage mechanism of the BPOE at discharge process. (a)p-undoping for the discharge process (at the potential above the initial OCV) of the BPOE. Electrons are extracted from the anode and are injected into the BPOE. Both anion (ClO4−) and cation (Na+) will travel back to the electrolyte during thep-undoping discharge process to maintain electrical neutrality. (b)n-doping for the discharge process (at the potential below the initial OCV) of the BPOE. Electrons are extracted from the anode and are injected into the BPOE. Na+will be doped into the BPOE during then-doping discharge process to maintain electrical neutrality. (c) Summary of the discharge process of energy storage device using a BPOE, which is linearly, continuously connectedp-dopable andn-dopable region. The total specific energyEtotal(Wh kg−1) can be calculated by summing the specific energy obtained duringp-undopingEp-undoping(Wh kg−1), indicated by the red area, and the specific energy obtained duringn-dopingEn-doping(Wh kg−1), indicated by the blue area.Etotal=Ep-undoping+En-dopingcan be calculated by:Etotal=whereQ(t) (mAh g−1)=constant current densityI0(mA g−1) ×t(h), is the specific capacity,t(h) is the discharge time andV(t) is the potential. Figure 5: Energy storage mechanism of the BPOE at discharge process. ( a ) p -undoping for the discharge process (at the potential above the initial OCV) of the BPOE. Electrons are extracted from the anode and are injected into the BPOE. Both anion (ClO 4 − ) and cation (Na + ) will travel back to the electrolyte during the p -undoping discharge process to maintain electrical neutrality. ( b ) n -doping for the discharge process (at the potential below the initial OCV) of the BPOE. Electrons are extracted from the anode and are injected into the BPOE. Na + will be doped into the BPOE during the n -doping discharge process to maintain electrical neutrality. ( c ) Summary of the discharge process of energy storage device using a BPOE, which is linearly, continuously connected p -dopable and n -dopable region. The total specific energy E total (Wh kg −1 ) can be calculated by summing the specific energy obtained during p -undoping E p-undoping (Wh kg −1 ), indicated by the red area, and the specific energy obtained during n -doping E n-doping (Wh kg −1 ), indicated by the blue area. E total = E p-undoping+ E n-doping can be calculated by: E total = where Q ( t ) (mAh g −1 )=constant current density I 0 (mA g −1 ) × t (h), is the specific capacity, t (h) is the discharge time and V ( t ) is the potential. Full size image The electrochemical property of the porous organic electrode in half-cells is compared with other proposed electrode materials in a Ragone plot ( Fig. 6a and Supplementary Fig. S6 ) and the round-trip energy efficiency ( Fig. 6b , Supplementary Figs S6 and S7 ). Our porous organic electrode exhibits a specific energy of ~500 Wh kg –1 and a specific power of 10 kW kg –1 ( Fig. 6a ); where the weight is based on the mass of BPOE. Promisingly, the volumetric energy is ~250 Wh L –1 (the density of the BPOE is 0.5108, g cm –3 ), which may compare favourably to lead−acid or Ni–Cd batteries with a specific volumetric energy of ~100 Wh L cell –1 in full cells. The volumetric energy (Wh L −1 ) of lead−acid and Ni−Cd in full cells is distributed around 100 Wh L cell −1 . Here the volumetric energy of the BPOE is ~250 Wh L −1 considering only the mass of the BPOE. If we assume that the volume of BPOE constitutes 40% of total volume of a sodium−organic energy storage device, this full cell will provide ~100 Wh L cell −1 , which is as good as for other rechargeable batteries, such as lead−acid and Ni−Cd batteries. This result is highly promising. For example, sodium–sulphur (NAS) batteries (indicated as a yellow region in Fig. 4a ) are a promising energy storage device for stationary electricity storage uses [4] , [8] . 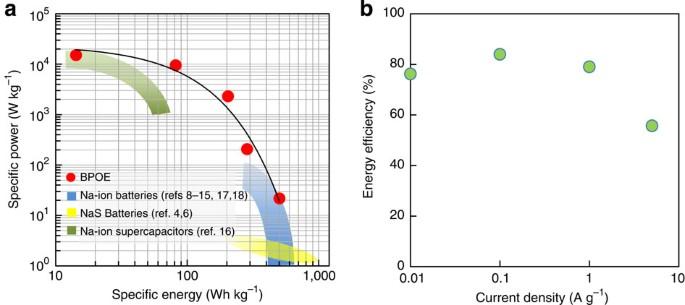Figure 6: Ragone plots and round-trip energy efficiency of sodium-organic energy storage device. (a) Ragone plots for a sodium-organic energy storage device using a BPOE and various sodium-based energy storage devices in half-cells. The specific energy was calculated on the basis of the half-cells using sodium metal as an anode. (b) Round-trip energy efficiency of the sodium-organic energy storage device. NAS batteries have a theoretical specific energy of 975 Wh kg –1 for the following reactions (equation (3), a theoretical specific capacity of 487 mAh g –1 with an average cell voltage of ~2 V): Figure 6: Ragone plots and round-trip energy efficiency of sodium-organic energy storage device. ( a ) Ragone plots for a sodium-organic energy storage device using a BPOE and various sodium-based energy storage devices in half-cells. The specific energy was calculated on the basis of the half-cells using sodium metal as an anode. ( b ) Round-trip energy efficiency of the sodium-organic energy storage device. Full size image However, this system has safety problems due to its high operation temperature of 300–350 °C ( [8] ). Indeed, full cells can provide much less specific energy due to limited practical cell configurations related to this safety problem. In contrast, we can operate the porous organic electrode at room-temperature with a specific energy comparable to NAS batteries. Also, this system shows a longer cycle life of 7,000 cycles compared with 4,500 cycles for NAS batteries and the energy efficiency of the BPOE is ~80% ( Fig. 6b ), which is comparable to 85% of NAS batteries [8] , and higher than ~70% of redox-flow batteries [55] , but the self-discharge characteristic of the NAS and sodium-ion batteries based on the intercalation mechanism are better than for the BPOE electrodes ( Supplementary Fig. S8 ). These issues could be improved by optimization of electrode assembly processes and further fundamental investigations of the BPOE, especially on the energy storage mechanism. The key point is that the porous organic electrode has a remarkably high-specific power of 10 kW kg –1 ; a performance not yet reached in Na-ion batteries. These properties of the BPOE are comparable to O3-type NaNi 0.5 Mn 0.5 O 2 (ref. 16 ) and P2-type Na x [Fe 1/2 Mn 1/2 ]O 2 (ref. 6 ), which are performed as state-of-the-art high-performance cathodes for Na-ion batteries, and are much higher than for other intercalation compounds such as fluorophosphates [12] , [13] , NASICONs [14] and olivines [15] . By combing state-of-the-arts anodes [27] , [56] , [57] , and electrolytes, such as ionic liquids [58] or NaPF 6 in EC:PC (ref. 59 ), the safety problem, which is one of the most important points for any practical technology, of a sodium-organic energy storage device could be improved. In summary, we have demonstrated the excellent electrochemical performance of a porous organic electrode for sodium-based energy storage devices with even compared with other sodium battery systems, and it is, therefore, a promising material for next-generation energy storage devices. This is, to the best our knowledge, the first report of a high-performance sodium-based energy storage device using an organic cathode. BPOEs are a new material platform to develop alternative, high-performance rechargeable energy storage devices by using cost-effective and abundant organic materials. Synthesis of the porous organic electrode The BPOE was synthesized by ionothermal synthesis [30] ; heating a mixture of p -dicyanobenzene and ZnCl 2 in quartz ampules at 400 °C for 40 h. The obtained samples were washed with 1 M HCl and distilled water for several times. After drying, we used this material as the BPOE without further treatments. The conductivity of the as-prepared BPOE was 4.09 × 10 −6 S cm −1 at 25 °C, which agrees well with the values for non-doped conjugated polymers [60] . The conductivity was measured by the impedance spectroscopy technique (see Supplementary Discussion ). We used steel electrodes and held a pellet of the as-prepared BPOE by using them to measure the impedance spectroscopy response. A frequency range from 10 mHz to 10 kHz with an amplitude of 500 mV was applied. Physical characterizations The electron energy-loss spectroscopy measurements were carried out using a Tecnai F30 (FEI company, equipped with a Gatan GIF 200 imaging energy filter) operated at an acceleration voltage of 300 kV by using a special sample holder, which can keep the organic specimen cool. The FT-IR measurement was carried out by using a FT-IR-6200 (JASCO) with KBr-IR measurements. The RSMs were carried out by using a Ventuno (NSR-1000DT, JASCO) with a laser excitation of 632.8 nm from a He-Ne laser. We have prepared samples for the spectroscopic measurements by the following method: the electrochemical doping of ClO 4 − in the BPOE was carried out by using galvanostatic intermittent titration technique. After the electrochemically doping, the doped BPOE was washed by PC and measured the Raman spectra. The powder X-ray diffraction measurement was carried out on a Stadi P (STOE) diffractometer using Cu Kα 1 radiation. The nitrogen physisorption measurements were carried out at 77 K up to 1 bar using a Quantachrome Autosorb 1C apparatus. Pore size distribution was obtained by applying the QS-DFT equilibrium model for nitrogen on carbon with slit pores at 77 K. Electrochemical characterization Electrodes were made by mixing active material (70 wt.%), carbon (carbon black; 20 wt.%), and binder (carboxyl methyl cellulose; 10 wt.%). We used Al current collectors. The loading mass was ~1.5 mg cm −2 and the electrode thickness was ~100 μm. We assembled the cells in a purge-type dry glove box (MIWA MFG) filled with high purity Ar gas (N50=99.999%) and tested them on a multichannel potentiostatic-galvanostatic system (SD-8, Hokuto-denko) and a frequency response analyser (SI 1250, Solatron). We used sodium metal as an anode and a reference electrode. We used 1 M NaClO 4 in propylene carbonate (Kishida Chemicals) as an electrolyte and in a three-electrode beaker cell as the test cell. The charge–discharge properties were recorded in a potential range from 4.1 to 1.3 V versus Na/Na + . EIS measurements were carried out at 3.3 V versus Na/Na + ( p -dopable region) and 2.3 V versus Na/Na + ( n -dopable region) after achieving each quasi-equilibrium state by taking a rest of 1 h after the doping. A frequency range from 10 mHz to 10 kHz with an amplitude of 10 mV was applied for the EIS measurements. The fitting was carried out by using Z-View (Scribner Associates). We have measured all charge–discharge properties after charging till 4.1 V versus Na/Na + ( p -doped state of the BPOE). Calculation of specific power ( P ) and specific energy ( E ) Specific energy E (Wh kg −1 ) can be calculated by E = where t cut (hour) is a discharge time, I 0 (A) is a constant current, m (kg) is a mass of the active material, and V ( t ) is a time-dependent voltage in the dimension of V. Specific power P (W kg −1 ) can be calculated by P = E / t cut . Also see Supplementary Figs S6, S7 . How to cite this article: Sakaushi, K. et al . Aromatic porous-honeycomb electrodes for a sodium-organic energy storage device. Nat. Commun. 4:1485 doi: 10.1038/ncomms2481 (2013).